Directing reaction pathways by catalyst active-site selection using self-assembled monolayers One key route for controlling reaction selectivity in heterogeneous catalysis is to prepare catalysts that exhibit only specific types of sites required for desired product formation. Here we show that alkanethiolate self-assembled monolayers with varying surface densities can be used to tune selectivity to desired hydrogenation and hydrodeoxygenation products during the reaction of furfural on supported palladium catalysts. Vibrational spectroscopic studies demonstrate that the selectivity improvement is achieved by controlling the availability of specific sites for the hydrogenation of furfural on supported palladium catalysts through the selection of an appropriate alkanethiolate. Increasing self-assembled monolayer density by controlling the steric bulk of the organic tail ligand restricts adsorption on terrace sites and dramatically increases selectivity to desired products furfuryl alcohol and methylfuran. This technique of active-site selection simultaneously serves both to enhance selectivity and provide insight into the reaction mechanism. Furfurals are important platform chemicals produced from biomass feedstocks by dehydration of simple sugars [1] , [2] and serve as important model compounds for multifunctional molecules. These highly reactive molecules represent a classic example of the challenge of selectivity in heterogeneous catalysis, as they interact with catalytic surfaces through all of their functional groups, resulting in a diverse range of products. In particular, on noble metal catalysts under hydrogenation conditions, the aromatic furan ring has a tendency to adsorb strongly on the surface, resulting in decarbonylation (DC) and ring hydrogenation (RH) to produce furan and tetrahydrofuran (THF) as the dominant reaction products. Conversely, reaction steps such as aldehyde hydrogenation (AH) and hydrodeoxygenation (HDO) necessary for conversion of furfuryl oxygenates to desirable fuels (furfuryl alcohol and methylfuran) do not occur as readily. 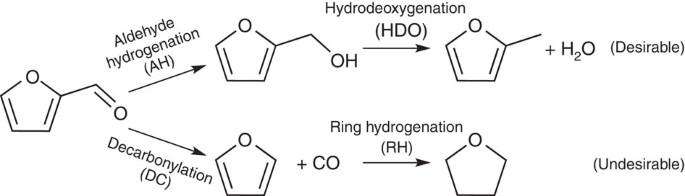Figure 1: Reaction pathways. Furfural hydrogenation. [3] , [4] , [5] , [6] , [7] , [8] Figure 1 depicts the major reaction pathways for furfural hydrogenation. Figure 1: Reaction pathways. Furfural hydrogenation. Full size image A number of techniques have been used to control reaction selectivity by the use of surface modifiers. Carbon monoxide is well known as a surface poison that can reduce surface ensemble size to control selectivity [9] , [10] but must continuously be added to the system at reaction temperatures, and the coverage/packing cannot be readily controlled. Organic modifiers such as thiophene [11] have been added to enhance selectivity, but creating a consistent surface remains a challenge because of inconsistencies arising from different preparation techniques. Even in studies where the same modifier and preparation techniques were used, dramatic differences have been reported [12] presumably because of subtle differences in the final modifier state. Although these approaches may improve catalytic performance in specific cases, it is important to develop a technique to systematically and reproducibly control the catalyst near-surface environment. Self-assembled monolayers (SAMs) have recently been utilized as modifiers to control reactivity in heterogeneous catalysis [13] , [14] , [15] , [16] , [17] , [18] . SAMs are attractive modifiers because they form ordered overlayers, and their chemistry (and thus their effect on surface reactivity) can be tuned by changing the molecular structure of the organic ‘tail’ function. For example, altering the surface density of alkanethiolate SAM modifiers by altering the steric bulk of the tail function has been shown to dramatically affect reactivity for several reactants by controlling the availability of different active sites on supported Pd/Al 2 O 3 catalysts [19] . However, the manipulation of SAM sterics for controlling reaction selectivity has not previously been demonstrated. Here we report the ability of controlled modifier density to direct furfural hydrogenation along a desired reaction pathway using SAMs formed from octadecanethiol (C18), which forms a dense (√3 × √3)R30 adsorption geometry with a nearest neighbour distance of ~ 4.7 Å on Pd fcc(111) surfaces [20] , or 1-adamantanethiol (AT), which forms a sparse (7 × 7) unit cell structure [21] with a nearest neighbour distance of ~ 6.4 Å, to coat supported Pd/Al 2 O 3 catalysts. Measurements of furfural hydrogenation kinetics were performed in conjunction with infrared spectroscopy to provide insight into the principles of active-site selection for the production of the valuable products methylfuran and furfuryl alcohol, as opposed to the less desirable furan and THF. Catalytic reactions Gas-phase hydrogenation of furfural was conducted over 5 and 1 wt% Pd/Al 2 O 3 catalysts in a tubular packed bed flow reactor at atmospheric pressure. Transmission electron microscopy (TEM) was used to determine the average size of the supported Pd particles, 6 and 3 nm ( Supplementary Figs S1 and S2 ), for the 5 and 1 wt% catalysts, respectively. As shown in Fig. 2 , using uncoated Pd catalysts, the dominant product was furan, and the rate of DC was about two orders of magnitude higher than that of aldehyde hydrogenation (AH) and HDO. Accordingly, the selectivity towards the desirable products, furfuryl alcohol and methylfuran, was negligible using the uncoated Pd catalyst. When the catalysts were modified with the sparsely packed AT SAM, there was a minor enhancement in selectivity towards the desired products, although selectivity to furan was still high. Notably, the densely coated C18 catalysts exhibited a dramatic improvement in selectivity towards the desired products. In particular, the C18-coated 1 wt% Pd/Al 2 O 3 catalyst exhibited over 55% selectivity to furfuryl alcohol and 35% selectivity to methylfuran. As methylfuran is produced in a series reaction from furfuryl alcohol, its selectivity can be improved to >70% even on the C18-coated 5% Pd/Al 2 O 3 catalyst at higher conversion (see Supplementary Table S1 ). 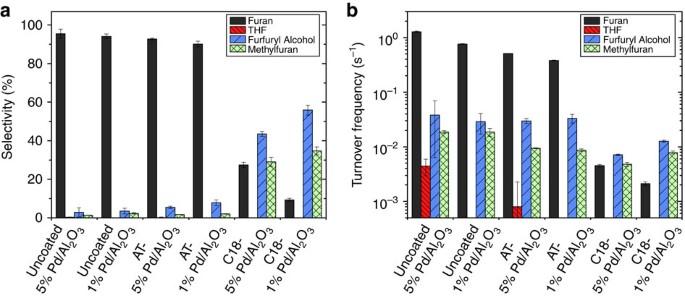Figure 2: Gas-phase hydrogenation of furfural. (a) Product selectivity for furfural hydrogenation over uncoated and alkanethiolate SAM-coated Pd/Al2O3catalysts. (b) Rate of production normalized by number of surface sites on the uncoated catalyst. Hydrogenations were carried out continuously at 190 °C at a 25:1 molar ratio of H2to furfural. Selectivity and rate are reported at 13±2% conversion of furfural fed. Error bars indicate the s.d. of 12 repeated measurements of product concentration. Figure 2: Gas-phase hydrogenation of furfural. ( a ) Product selectivity for furfural hydrogenation over uncoated and alkanethiolate SAM-coated Pd/Al 2 O 3 catalysts. ( b ) Rate of production normalized by number of surface sites on the uncoated catalyst. Hydrogenations were carried out continuously at 190 °C at a 25:1 molar ratio of H 2 to furfural. Selectivity and rate are reported at 13±2% conversion of furfural fed. Error bars indicate the s.d. of 12 repeated measurements of product concentration. Full size image Importantly, although the overall rate of reaction was decreased by the SAM coatings, as expected, this decrease was nearly completely attributed to the undesirable DC pathway (see Fig. 2b ). As the SAM packing became increasingly dense, the rate of DC decreased by three orders of magnitude. However, the rates of aldehyde hydrogenation and HDO were nearly unaffected. Thus, the increase in selectivity to the desired products was not because of an increase in the rate of the desired reaction but rather because of inhibition of the undesired reaction. In previous work, we found that adsorption on catalyst terrace sites was reduced systematically with increasing thiol SAM density, whereas adsorption on step edges and defects was mostly unaffected [19] . We therefore hypothesized that the reduction in the rate of DC on the thiol-modified catalysts was a direct effect of limiting access to terrace sites. Supporting this notion, single-crystal studies of benzyl alcohol and benzaldehyde (functionally similar to furfural) on Pd(111) have shown that DC to produce benzene is dominant when the molecules can adopt a flat-lying conformation [22] . In addition, density functional theory calculations show that the furan ring in furfural preferentially adsorbs in a threefold hollow site for flat-lying structures [7] , [8] , [23] . Thus, we expect that DC and RH occur primarily on threefold terrace sites where a large contiguous ensemble of sites is available. In the case of furfural, the high selectivity to furan on both the uncoated and AT-modified catalysts suggested that the ensemble requirement for DC was satisfied on these catalysts but not on the C18-modified catalyst. As the rates of furfuryl alcohol and methylfuran production were unaffected on the coated catalysts, we hypothesize that these products were formed primarily at the step edge and defect sites. Identification of adsorption sites by infrared spectroscopy To directly test the availability of specific adsorption sites, diffuse reflectance Fourier transform infrared spectroscopy (DRIFTS) was performed under variable pressures of carbon monoxide; in these experiments, peak positions are readily attributed to CO binding in threefold, bridging and top sites [24] . We previously found that on unmodified 5 wt% catalyst, increasing thiol density restricted adsorption on terrace sites ( Fig. 3a adapted from ref. 19 ). On the more crowded C18-coated catalysts, CO adsorbed only on threefold hollow (1,885 cm −1 ) and top sites at step edges and defects (2,051 cm −1 ). On AT-coated catalysts, CO had additional access to adsorption on terrace bridging (1,919 cm −1 ) and an additional type of linear (2,077 cm −1 ) sites on terraces. 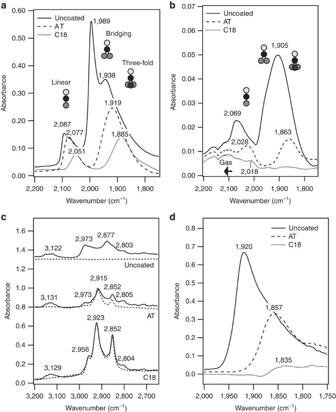Figure 3: DRIFT spectra for uncoated and SAM-coated catalysts. CO stretch region for uncoated and alkanethiolate SAM-coated (a) 5 wt% (adapted from ref.19) and (b) 1 wt% Pd/Al2O3catalysts. For linear adsorption on top sites, the lower wavenumber features are associated with adsorption at steps and edges, whereas higher wavenumber features are indicative of adsorption on terrace sites25. DRIFT spectra for samples after furfural exposure: (c) Hydrocarbon-stretching region for uncoated, AT and C18 catalysts. Dashed and solid lines are shown for samples before and after exposure, respectively. (d) CO production on the uncoated, AT and C18 catalysts after exposure to furfural. Figure 3: DRIFT spectra for uncoated and SAM-coated catalysts. CO stretch region for uncoated and alkanethiolate SAM-coated ( a ) 5 wt% (adapted from ref. 19 ) and ( b ) 1 wt% Pd/Al 2 O 3 catalysts. For linear adsorption on top sites, the lower wavenumber features are associated with adsorption at steps and edges, whereas higher wavenumber features are indicative of adsorption on terrace sites [25] . DRIFT spectra for samples after furfural exposure: ( c ) Hydrocarbon-stretching region for uncoated, AT and C18 catalysts. Dashed and solid lines are shown for samples before and after exposure, respectively. ( d ) CO production on the uncoated, AT and C18 catalysts after exposure to furfural. Full size image The C18-modified 1 wt% particles inhibited furan production more than the same coating on the 5 wt% catalysts ( Fig. 2 ). Thus, if production of furan requires an ensemble of terrace sites, we would expect to see limited terrace CO adsorption on C18-modified 1 wt% catalysts. Figure 3b shows the DRIFT spectra for the modified and unmodified 1 wt% catalysts. The major peaks at 1,905 and 1,863 cm −1 on the uncoated and AT catalysts, respectively, were attributed to CO binding primarily on threefold terrace sites. The smaller peak area for this feature on the AT catalyst indicated reduced adsorption at terraces. On the C18 catalyst, this feature was essentially non-existent, supporting the hypothesis that the crowded monolayer on these smaller particles limited the availability of terrace sites. In contrast, the feature at 2,018 cm −1 was attributed to linear adsorption primarily at steps and edges. This feature was also present on the uncoated 1% catalyst at low pressures but was obscured at higher pressure by species adsorbed linearly on terrace sites (see Supplementary Fig. S3 for low CO pressure spectra). The peaks above 2,100 cm −1 were due to gas-phase CO, indicating that the catalysts were saturated with CO. As the rates of production of furfuryl alcohol and methylfuran were nearly the same on all the catalysts and the availability of step and edge sites was mostly unaffected by the thiol modifiers, we suggest that the production of these species occurs preferentially at these sites, whereas furan production probably requires terrace sites. The dearth of threefold hollow sites on the 1 wt% catalyst was presumably responsible for the absence of the THF product, as RH requires a large number of contiguous surface sites [26] , [27] allowing the ring to lie flat. The proposed adsorption mechanism is depicted in Fig. 4 . 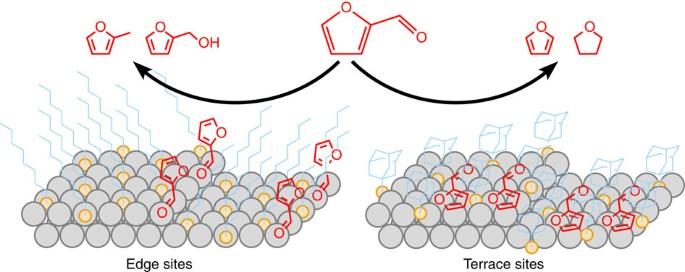Figure 4: Proposed schematic depicting active-site selection. On C18-modified surfaces furfural binds upright on step edges and defects, whereas on AT-modified surfaces furfural can lie flat on a terrace. Figure 4: Proposed schematic depicting active-site selection. On C18-modified surfaces furfural binds upright on step edges and defects, whereas on AT-modified surfaces furfural can lie flat on a terrace. Full size image In situ DRIFT spectroscopy during exposure to furfural on modified and unmodified catalysts provided further evidence for reduced DC and decomposition on the more crowded surfaces. C18, AT and unmodified 5 wt% Pd/Al 2 O 3 were each exposed to ~ 60 (mg furfural fed)/(mg Pd × h) for 20 min using He carrier gas. Spectra were collected after removing the gas-phase furfural but still under the flow of He (see Fig. 3c ). The dashed spectra show the catalyst before exposure to furfural for the uncoated, AT and C18 catalysts. Before exposure, both C18- and AT-modified catalysts exhibited spectral features associated with an ordered monolayer, where the asymmetric methylene stretches were observed at 2,923 and 2,915 cm −1 for C18 and AT, respectively. This is compared with fcc(111) surfaces where these peaks were observed at 2,918 and 2,911 cm −1 , respectively [20] , [28] . In the case of C18, these positions are intermediate between crystalline (2,918 cm −1 ) and liquid-like (2,928 cm −1 ) [29] features for C18. The appearance of the broad C-H-stretching peaks between ~ 2,800 and 3,000 cm −1 on the uncoated catalyst indicated the production of decomposition intermediates bound to the catalyst. Single-crystal and density functional theory studies of furanic species on Pd(111) have attributed stretches in this range to a combination of CH and CH 2 containing fragments from adsorption of the furan ring and decomposition to surface hydrocarbon species [7] , [30] , [31] . The appearance of CH 2 stretches, not present in the parent furfural molecule, may be attributed to reaction of the adsorbed furan ring with surface hydrogen atoms produced from decomposition of neighbouring adsorbates. On the AT catalyst, the amount of furfural decomposition was significantly reduced; however, peaks at 2,852 and 2,973 cm −1 , similarly attributed to CH and CH 2 stretches, indicated some adsorption of the furan ring, consistent with the production of both furan and THF on this catalyst. On the C18 catalyst, there was essentially no production of decomposition products on the catalyst after furfural exposure. The appearance of the broad peak around ~ 3,130 cm −1 and the peak at ~ 2,805 cm −1 , present on all of the catalysts after furfural exposure, indicated the presence of the symmetric and asymmetric C-H stretches of the unsaturated furan ring and the aldehyde constituent, respectively. These stretches are also present in the spectrum of liquid-like furfural [32] , suggesting the presence of physisorbed or weakly chemisorbed furfural on all catalyst surfaces. Spectra obtained after exposure to furfural also provided direct information about the extent of DC ( Fig. 3d ) in the form of the presence of bound CO. The uncoated catalyst showed significant CO binding in both threefold and bridging sites (peak at 1,920 cm −1 ). CO production on the AT-modified catalyst occurred primarily on threefold sites and was reduced with respect to the uncoated catalyst. Minimal CO production occurred on the C18 catalyst, with a small amount formed at the threefold hollow sites, likely at defects in the SAM. Adsorption to these sites can be seen in the results of CO DRIFTS experiments on C18-modified 5 wt% Pd Al 2 O 3 but not the C18-modified 1 wt% Pd/Al 2 O 3 , consistent with the decreased rate of production of furan on the C18-modified 1 wt%. These results again support the kinetic data, demonstrating that DC is inhibited by increasing modifier crowding on the catalyst terraces. In summary, we have shown that alkanethiolate SAM-modified Pd catalysts increase the selectivity of furfural hydrogenation to furfuryl alcohol and methylfuran by limiting the availability of particular surface sites. By using a less dense SAM, such as one created by AT, a portion of the threefold terrace sites can be blocked and the rate of DC and RH decreased. Using a dense SAM, such as one created by octadecanethiol, access to the threefold sites can be severely limited, drastically reducing the rate of DC leading to selectivity enhancement for aldehyde hydrogenation and HDO. Thus, active-site selection using SAM modifiers in catalysis can potentially serve as an alternative (or complement) to recent efforts [33] , [34] , [35] , [36] aimed at modifying shape, and thus surface-site distribution, of supported metal nanoparticles to control selectivity. Materials Pd/Al 2 O 3 catalysts (5 and 1 wt%), 1-octadecanethiol (98%), AT (95%), furfural (99%) and 200-proof HPLC-grade ethanol were purchased from Sigma-Aldrich. Catalysts were used as received for uncoated reactions. Ultra-high purity H 2 and He were obtained from Airgas. SAM preparation and characterization AT and C18 SAMs were deposited on the catalysts by dissolving the thiol in 40 ml ethanol at a concentration of 4.25 mmol l −1 . The surface area of the less disperse 5 wt% Pd/Al 2 O 3 ( D =0.266) was ~ 2.7 × that of the more disperse 1 wt% Pd/Al 2 O 3 ( D =0.414) per mass of supported catalyst, as determined by TEM ( Supplementary Figs S1 and S2 ). Thus, 250 mg of 1 wt% Pd/Al 2 O 3 or 100 mg of 5 wt% Pd/Al 2 O 3 was added to the solution to expose a similar surface area of Pd to the thiol solution. The catalysts were allowed to settle for at least 12 h. The supernatant was decanted, and 40 ml ethanol was added to wash off any excess thiol that had not adsorbed. The catalysts were allowed to settle for an additional 2 h, and then the supernatant was decanted. The catalysts were allowed to dry in air before use. The sulphur content was analysed using inductively coupled plasma-atomic emission spectrometry. The results demonstrated that there was 2.1 × the amount of sulphur present on the C18 catalysts than that on the AT catalysts, which is approximately the amount expected from differences in coverage on single-crystal surfaces (~ 1.8 × more molecules for the C18 surface [20] , [21] ). No sulphur adsorption was found on pure Al 2 O 3 . In addition, an approximate thiolate concentration was inferred from the hydrocarbon-stretching region of the freshly modified catalysts. With 18 carbons for C18 and 10 for AT, the total hydrocarbon peak area was nominally expected to be ~ 3.3 × greater for the C18 catalyst, taking into account the 1.8 × difference in coverage. Actual peaks from Fig. 3 showed ~ 3.7 × greater areas, indicating a more densely packed monolayer for the C18 than AT. Although the overall packing density of the C18 SAM was higher, defects were almost certainly present. Overall, the C18- and AT-modified catalysts exhibited features associated with an ordered monolayer where the asymmetric methylene stretches were observed at 2,923 and 2,915 cm −1 for each catalyst coating, respectively. This is compared with fcc(111) surfaces where these peaks were observed at 2,918 and 2,911 cm −1 , respectively [20] , [28] . Catalytic reactions Hydrogenations were conducted in a tubular packed bed flow reactor at 190 °C and atmospheric pressure. Helium was bubbled through furfural (Sigma-Aldrich) to achieve furfural gas-phase concentration y furfural =0.016 and mixed with H 2 at a 25:1 molar ratio of H 2 to furfural. The amount of catalyst used was varied systematically to achieve a conversion of 13±2% in all cases; weight hourly space velocities are listed in Supplementary Table S2 . Each reaction was run for at least 200 min; selectivity and conversion at the end of this period are reported here. Additional reactions were performed varying temperature and conversion to demonstrate the sequential nature of the reaction; as conversion increased, more methylfuran was produced relative to furfuryl alcohol and vice versa for decreased conversion ( Supplementary Table S1 ), indicating that reaction selectivity could be tuned using conversion. Representative kinetic plots showing selectivity and conversion as a function of time on stream ( Supplementary Fig. S4 ) reveal that over the course of the reaction, the uncoated catalyst experiences continuously decreasing activity. Conversely, the C18-coated catalyst exhibits constant conversion, showing that the SAMs are mostly stable under reaction conditions. Additional reactions were performed using the uncoated and C18-coated 5 wt% Pd/Al 2 O 3 , allowing the reaction to proceed for at least 15 h to further examine the stability of selectivity, conversion and SAM coating ( Supplementary Fig. S5 ). Comparison of reaction selectivity at 4 and 15 h shows no significant increase in the selectivity to furan for the C18-coated catalyst but a drop in conversion from 12 to 5%. DRIFT spectra before and after 15 h of reaction reveal a 3- and 5-cm −1 shift in the peak positions for asymmetric and symmetric methylene stretching, respectively. These data indicated some disordering of the monolayer, possibly because of the generation of gauche defects [20] . Importantly, the SAM was still present on the surface under reaction conditions at the time that selectivity and rates are reported. For stable operation over longer reaction times, it may be desirable to pursue approaches such as post-assembly crosslinking of SAMs [37] . The gas mixture passed over the catalyst and the reactor effluent was analysed using an Agilent Technologies 7890A gas chromatograph equipped with a 30 × 0.320 mm 2 Agilent HP-5 capillary column and flame ionization detector (split ratio=25:1, column flow rate=2 ml min −1 , oven temperature=50 °C). A representative gas chromatograph is shown in Supplementary Fig. S6 . Turnover frequencies for individual products reported in Fig. 2b are calculated by dividing the product flow rates by the number of surface sites on unmodified catalyst, based on the size of the metal particles and mass of catalyst used. Fourier transform infrared analysis Fourier transform infrared analysis was performed using a Thermo Scientific Nicolet 6700 FT-IR with a closed cell attachment (Harrick) for DRIFTS. Fifty scans at 4 cm −1 resolution were used for each spectrum. The quality of all coated samples was characterized in the C-H-stretching region (2,800–3,000 cm −1 ) to confirm monolayer formation before catalytic testing. For CO DRIFT experiments, catalyst samples were placed in a gastight cell that was evacuated to achieve an initial baseline pressure of <0.10 Torr. The 1% catalysts were determined to have ~ 2.7 × fewer active sites per gram of supported catalyst (as determined by TEM imaging), which resulted in an overall weaker signal intensity in the DRIFT spectra ( Fig. 3b ). In addition, the signal was further weakened because a reduced sample mass was loaded into the sample cup because of the lower density of the alumina support for the 1% Pd/Al 2 O 3 catalyst. Differences in the apparent density of the alumina support were determined to be ~ 3 × . TEM images confirm a more porous Al 2 O 3 support morphology for the 1% catalysts ( Supplementary Figs S1 and S2 ). This resulted in a weaker signal on the 1% catalyst than on the 5% catalyst (~ 8 × ). How to cite this article: Pang, S. H. et al . Directing reaction pathways by catalyst active-site selection using self-assembled monolayers. Nat. Commun. 4:2448 doi: 10.1038/ncomms3448 (2013).